The acetylation of tau inhibits its function and promotes pathological tau aggregation The microtubule associated protein tau promotes neuronal survival through binding and stabilization of MTs. Phosphorylation regulates tau–microtubule interactions and hyperphosphorylation contributes to the aberrant formation of insoluble tau aggregates in Alzheimer's disease (AD) and related tauopathies 1 . However, other pathogenic post-translational tau modifications have not been well characterized. Here we demonstrate that tau acetylation inhibits tau function via impaired tau–microtubule interactions and promotes pathological tau aggregation. Mass spectrometry analysis identified specific lysine residues, including lysine 280 (K280) within the microtubule-binding motif as the major sites of tau acetylation. Immunohistochemical and biochemical studies of brains from tau transgenic mice and patients with AD and related tauopathies showed that acetylated tau pathology is specifically associated with insoluble, Thioflavin-positive tau aggregates. Thus, tau K280 acetylation in our studies was only detected in diseased tissue, suggesting it may have a role in pathological tau transformation. This study suggests that tau K280 acetylation is a potential target for drug discovery and biomarker development for AD and related tauopathies. Tau proteins are expressed primarily in the central nervous system where the critical functions of promoting microtubule (MT) assembly and stability are mediated by six tau isoforms generated by mRNA alternative splicing containing either three (3R-tau) or four (4R-tau) MT-binding repeats [2] , [3] . Regulation of tau binding to MTs is mediated by serine/threonine phosphorylation, which decreases tau–MT-binding affinity [4] , [5] , [6] . However, aberrant accumulation of unbound hyperphosphorylated insoluble tau as neurofibrillary tangles (NFTs) is implicated in the pathogenesis of neurodegenerative tauopathies including Alzheimer's disease (AD; for review see refs 1 , 7 ). Genetic studies demonstrated that missense mutations that alter tau binding and MT assembly (for example, ΔK280, V337M, P301L, R406W) are pathogenic for frontotemporal dementia and parkinsonism linked to chromosome 17 (FTDP-17), which is characterized by prominent NFTs and neurodegeneration [8] , [9] , [10] , [11] . The mechanism leading normal soluble tau to become hyperphosphorylated and disengaged from MTs to form tau inclusions remains unknown and post-translational modifications other than phosphorylation could regulate tau function and aggregation. Notably, reversible lysine acetylation has emerged as a potential regulatory modification implicated in AD and other neurodegenerative disorders, and a recent study demonstrated that tau is modified by lysine acetylation [12] . However, the functional significance and implications of tau acetylation in neurodegenerative tauopathies are not clear. Thus, to determine whether tau acetylation is linked to tau aggregation and disease pathogenesis, we assessed tau acetylation in vitro , in cell-based models, in tau Tg mouse models, and in a wide spectrum of human tauopathies including AD. We provide evidence that tau acetylation at specific lysine residues impairs tau-mediated stabilization of MTs and enhances tau aggregation. Furthermore, tau acetylation is associated with insoluble, Thioflavin-positive NFTs in tau Tg mouse models and human tauopathies, implicating tau acetylation as a potential factor in the pathogenesis of neurodegenerative tauopathies. Acetylation impairs tau function and promotes tau fibrillization To fully characterize tau acetylation, recombinant full-length tau (T40) or a fragment encompassing all four MT-binding repeats (K18), were incubated with [ 14 C]-acetyl Co-A in the presence of the acetyltransferase Creb-binding protein (CBP) [13] . Although tau-K18 and tau-T40 displayed low-level auto-acetylation frequently seen with high-affinity substrates, CBP enhanced the acetylation of both full-length T40 and the K18 fragment, suggesting acetylated lysine residues lie within the MT-binding region ( Fig. 1a ). Tau-T40 was fibrillized in vitro to generate tau fibrils in which the MT-binding region forms the fibril core. These tau fibrils could not be acetylated indicating lysine residues are not accessible to acetylation in fibrillized tau. To confirm tau acetylation in vitro , immunoblotting using a pan-anti-acetyl-lysine antibody revealed that both T40 and K18 were acetylated in the presence of CBP ( Fig. 1b ). To assess the significance of tau acetylation, we determined the ability of acetylated tau-K18 ( Fig. 1c ) or full-length tau-T40 ( Supplementary Fig. S1 ) proteins to promote MT assembly using a light-scattering technique [8] . As expected, native K18 promoted tubulin assembly into MTs as determined by absorbance at 350 nm. In contrast, acetylated K18 failed to promote MT assembly, similar to the negative control K18 containing the K311D mutation, previously shown to impair tau–MT interactions [14] , [15] . 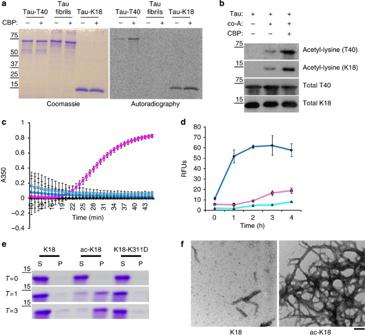Figure 1: Tau acetylation impairs MT assembly and promotes tau fibrillizationin vitro. (a) Recombinant full-length T40, 4R-tau MT-binding domain K18, or tau fibrils (seeMethodsfor fibrillization assay) were acetylated by incubation with [14C]-labeled acetyl-CoA in the presence or absence of CBP. Reaction products were analysed by SDS–PAGE and Coomassie blue staining followed by overnight radiographic exposure using STORM phosphor-imager software. (b) T40 or K18 proteins were incubated with acetyl-CoA and/or recombinant CBP and reaction products were subjected to immunoblot analysis using a polyclonal anti-tau-specific antibody for MT repeat domain (E10) and an anti-acetyl-lysine antibody. (c) MT assembly activities of K18 proteins were evaluated in light-scattering assays. Tubulin monomers (30 μM) were mixed with 40 μM tau proteins in MT assembly buffer supplemented with 2 mM guanosine triphosphate. MT assembly was determined by monitoring absorbance every minute at 350 nm using a SpectraMax plate reader. Colour key is as follows: native unmodified K18 (pink squares), acetylated K18 (blue triangles), K18 containing K311D mutation (turquoise X's) and no tau control (black diamonds). (d) Tau proteins (10 μM) were evaluated in fibrillization reactions using 10 μM heparin to induce assembly. At each time point, samples were incubated with 12.5 μM ThT and excitation/emission wavelengths were set to 450 and 510 nm, respectively. Colour key is as follows: native unmodified K18 (pink squares), acetylated K18 (blue diamonds) and K18-containing K311D mutation (turquoise triangles). Both MT assembly and fibrillization reactions were confirmed fromn=4 independent experiments. Error bars indicate standard error of the mean. (e) Tau proteins at indicated fibrillization time points (T=0, 1, 3 h) were centrifuged at 100,000gfor 30 min to generate a pellet fraction (P) containing tau fibrils and supernatants (S) containing unassembled tau protein. Samples were analysed by SDS–PAGE and Coomassie staining to monitor fibril formation. (f) Four-hour time points from fibrillization reactions were analysed by negative-staining EM. Note, at the concentration of 10 μM, native K18 did not fibrillize, whereas acetylated K18 had fibrillized extensively with morphologies similar to AD-like PHFs. Scale bar, 200 nm. Figure 1: Tau acetylation impairs MT assembly and promotes tau fibrillization in vitro . ( a ) Recombinant full-length T40, 4R-tau MT-binding domain K18, or tau fibrils (see Methods for fibrillization assay) were acetylated by incubation with [ 14 C]-labeled acetyl-CoA in the presence or absence of CBP. Reaction products were analysed by SDS–PAGE and Coomassie blue staining followed by overnight radiographic exposure using STORM phosphor-imager software. ( b ) T40 or K18 proteins were incubated with acetyl-CoA and/or recombinant CBP and reaction products were subjected to immunoblot analysis using a polyclonal anti-tau-specific antibody for MT repeat domain (E10) and an anti-acetyl-lysine antibody. ( c ) MT assembly activities of K18 proteins were evaluated in light-scattering assays. Tubulin monomers (30 μM) were mixed with 40 μM tau proteins in MT assembly buffer supplemented with 2 mM guanosine triphosphate. MT assembly was determined by monitoring absorbance every minute at 350 nm using a SpectraMax plate reader. Colour key is as follows: native unmodified K18 (pink squares), acetylated K18 (blue triangles), K18 containing K311D mutation (turquoise X's) and no tau control (black diamonds). ( d ) Tau proteins (10 μM) were evaluated in fibrillization reactions using 10 μM heparin to induce assembly. At each time point, samples were incubated with 12.5 μM ThT and excitation/emission wavelengths were set to 450 and 510 nm, respectively. Colour key is as follows: native unmodified K18 (pink squares), acetylated K18 (blue diamonds) and K18-containing K311D mutation (turquoise triangles). Both MT assembly and fibrillization reactions were confirmed from n =4 independent experiments. Error bars indicate standard error of the mean. ( e ) Tau proteins at indicated fibrillization time points ( T =0, 1, 3 h) were centrifuged at 100,000 g for 30 min to generate a pellet fraction (P) containing tau fibrils and supernatants (S) containing unassembled tau protein. Samples were analysed by SDS–PAGE and Coomassie staining to monitor fibril formation. ( f ) Four-hour time points from fibrillization reactions were analysed by negative-staining EM. Note, at the concentration of 10 μM, native K18 did not fibrillize, whereas acetylated K18 had fibrillized extensively with morphologies similar to AD-like PHFs. Scale bar, 200 nm. Full size image In addition to promoting MT assembly, the MT repeat domain is the core region required for tau fibrillization into AD paired helical filaments (PHFs) and straight filaments found in other tauopathies [16] , [17] . Given the robust tau acetylation within the MT-binding region, we determined whether acetylation of tau-K18 ( Fig. 1d ) or tau-T40 ( Supplementary Fig. S1 ) affects tau fibrillization. Using a heparin-induced tau fibrillization assay quantified by Thioflavin-T (ThT) binding, native K18 did not fibrillize during the 4-h incubation period, whereas acetylated K18 fibrillized rapidly by 3 h indicating acetylation enhanced the K18 fibrillization rate ( Fig. 1d ). Similar enhancement of tau-T40 aggregation was also observed ( Supplementary Fig. S1 ). Sedimentation analysis of acetylated K18 confirmed this finding and showed significant fibril accumulation in pellet fractions from 1 to 3 h, whereas native K18 was predominantly in the supernatant fraction ( Fig. 1e ). As expected, the negative control K18-K311D mutant did not fibrillize using both ThT and sedimentation assays. Confirming these observations, negative staining electron microscopy (EM) showed that acetylated K18 but not native K18 formed abundant filaments after 4 h ( Fig. 1f ). Thus, acetylation of tau proteins in vitro not only impaired the ability of tau to promote MT assembly but also enhanced tau fibrillization, similar to tau harbouring MT-binding region mutations in several FTDP-17 kindreds [18] , [19] . To characterize tau acetylation in cells, doxycycline-inducible HEK-293 cells stably expressing full-length tau-T40 (HEK-T40 cells) were labelled with [ 3 H]-acetate followed by immunoprecipitation, SDS–PAGE and autoradiography ( Fig. 2a ). Although low-level tau acetylation was observed in untreated HEK-T40 cells, treatment with the pan histone deacetylase (HDAC) inhibitor trichostatin A (TSA), but not the Sir2 class inhibitor nicotinamide [20] , resulted in a dramatic increase in acetylated tau levels. To further confirm tau acetylation, tau was immunoprecipitated from HEK-T40 cells transiently transfected with CBP, and acetylated tau was detected using an anti-acetyl-lysine antibody ( Fig. 2b ). CBP transfection alone promoted detectable tau acetylation, however, CBP expression in combination with TSA treatment led to a dramatic accumulation of acetylated tau. Notably, acetylated tau can be modified by HDAC activity as co-expression of CBP with wild-type (WT) HDAC6, but not a catalytically dead HDAC6 mutant, resulted in tau deacetylation ( Fig. 2c ). Thus, tau is dynamically regulated by reversible acetylation and deacetylation reactions. 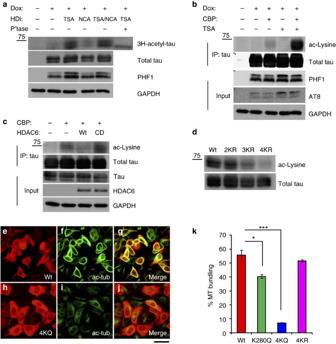Figure 2: Tau acetylation in cells inhibits tau-mediated MT stabilization. (a) Doxycycline (Dox)-treated HEK-T40 cells were cultured in the presence of either trichostatin A (TSA), nicotinamide (NCA) or both and pulse labelled with [3H]-acetate for 2 h. Tau was immunoprecipitated, treated with λ-phosphatase where indicated, and analysed by SDS–PAGE followed by autoradiography and exposure to film for 2 weeks. Total cellular lysates were immunoblotted using anti-tau (T14/T46), PHF-1 and GAPDH antibodies. (b) Cells transfected with CBP were treated with TSA and acetylated tau levels were determined by immunoprecipitation/immunoblot analysis using anti-acetylated lysine antibody. Cellular lysates were immunoblotted using T14/46, PHF-1, AT8 and GAPDH antibodies. (c) Cells were transfected with CBP and either wild-type (WT) HDAC6 or the catalytically dead (CD) HDAC6-H611A mutant and tau acetylation was determined by immunoblotting similar tobabove. (d) QBI-293 cells were transfected with WT T40, 2KR (K280/281R), 3KR (K163/280/281R) or 4KR (K163/280/281/369R) mutant T40 and cell lysates were immunoblotted using anti-acetyl-lysine and total tau (T14/T46) antibodies. (e–j) QBI-293 cells were transfected with WT T40 (e, red) and MT bundling was determined by immunofluorescence using anti-acetylated tubulin antibodies as shown for WT (f, green). Merged images indicate stabilized microtubules as shown for WT (g). QBI-293 cells were transfected with 4KQ (K163/280/281/369Q) (h, red) and MT bundling was determined by immunofluorescence using anti-acetylated tubulin antibodies as shown for 4KQ (i, green) and merged images (j). Representative images are shown fromn=4 independent experiments. Note, WT tau (e–g), but not 4KQ (h–j), promotes robust MT bundling. Scale bar, 50 μm. (k) QBI-293 cells were transfected with WT T40 (red bar), K280Q (green bar), 4KQ (K163/280/281/369Q) (blue bar) or 4KR (purple bar) mutant plasmids and MT bundling was determined from tau-expressing cells by quantification of ten fields/transfection and values are represented as %MT bundling from tau-expressing cells. Error bars indicate standard error of the mean. *Pvalue=0.006, ***Pvalue=8.46×10−6as determined by Student'st-test. Figure 2: Tau acetylation in cells inhibits tau-mediated MT stabilization. ( a ) Doxycycline (Dox)-treated HEK-T40 cells were cultured in the presence of either trichostatin A (TSA), nicotinamide (NCA) or both and pulse labelled with [ 3 H]-acetate for 2 h. Tau was immunoprecipitated, treated with λ-phosphatase where indicated, and analysed by SDS–PAGE followed by autoradiography and exposure to film for 2 weeks. Total cellular lysates were immunoblotted using anti-tau (T14/T46), PHF-1 and GAPDH antibodies. ( b ) Cells transfected with CBP were treated with TSA and acetylated tau levels were determined by immunoprecipitation/immunoblot analysis using anti-acetylated lysine antibody. Cellular lysates were immunoblotted using T14/46, PHF-1, AT8 and GAPDH antibodies. ( c ) Cells were transfected with CBP and either wild-type (WT) HDAC6 or the catalytically dead (CD) HDAC6-H611A mutant and tau acetylation was determined by immunoblotting similar to b above. ( d ) QBI-293 cells were transfected with WT T40, 2KR (K280/281R), 3KR (K163/280/281R) or 4KR (K163/280/281/369R) mutant T40 and cell lysates were immunoblotted using anti-acetyl-lysine and total tau (T14/T46) antibodies. ( e – j ) QBI-293 cells were transfected with WT T40 ( e , red) and MT bundling was determined by immunofluorescence using anti-acetylated tubulin antibodies as shown for WT ( f , green). Merged images indicate stabilized microtubules as shown for WT ( g ). QBI-293 cells were transfected with 4KQ (K163/280/281/369Q) ( h , red) and MT bundling was determined by immunofluorescence using anti-acetylated tubulin antibodies as shown for 4KQ ( i , green) and merged images ( j ). Representative images are shown from n =4 independent experiments. Note, WT tau ( e–g ), but not 4KQ ( h – j ), promotes robust MT bundling. Scale bar, 50 μm. ( k ) QBI-293 cells were transfected with WT T40 (red bar), K280Q (green bar), 4KQ (K163/280/281/369Q) (blue bar) or 4KR (purple bar) mutant plasmids and MT bundling was determined from tau-expressing cells by quantification of ten fields/transfection and values are represented as %MT bundling from tau-expressing cells. Error bars indicate standard error of the mean. * P value=0.006, *** P value=8.46×10 −6 as determined by Student's t -test. Full size image Identification and characterization of acetylated lysine residues in tau To identify acetylated lysine residues in tau, mass spectrometry analysis using nanoLC/nanospray/MS/MS was performed on recombinant T40 acetylated in vitro . Multiple lysine residues within the repeat region and adjacent proline-rich region showed significant acetylation ( Supplementary Table S1 , P value <0.05 significance score). To validate in vitro acetylated sites, CBP-transfected HEK-T40 cells were treated with TSA and immunoprecipitated tau protein bands were excised for mass spectrometry analysis ( Supplementary Fig. S2 and Supplementary Table S2 ). Significant acetylation was detected on the double lysine K280/K281 within the peptide V–Q–I–I–N–K–K in the second MT-binding repeat as well as K163 and K369 within the proline-rich region and MT-binding region, respectively (see Table 1 ). Western analysis of lysine→arginine mutants demonstrated that mutation of all four lysine residues (tau-4KR) dramatically reduced tau acetylation in cells, indicating that K163/280/281/369 represent the major sites of tau acetylation ( Fig. 2d ). Table 1 Tau acetylation sites identified by mass spectrometry. Full size table To evaluate the functional significance of tau acetylation, K→Q acetylation mimetic mutants were generated and expressed in HEK-293 cells. Consistent with previous reports [21] , WT tau overexpression stabilized MTs and promotes MT bundling, as detected by immunofluorescence (IF) using an anti-acetyl-tubulin antibody ( Fig. 2e–g ). However, expression of a tau-4KQ acetylation mimetic (K163/280/281/369Q), but not a tau-4KR non-mimetic mutant, showed a dramatic reduction in MT bundling activity (WT ∼ 55% versus 4KQ ∼ 7% versus 4KR ∼ 50% bundling), consistent with loss of tau function induced by acetylation ( Fig. 2h–j ). Interestingly, MT bundling observed with the single K280Q mimetic was significantly reduced ( ∼ 40% bundling), indicating acetylation of a single-lysine residue, that is, K280, is critical in regulating tau function ( Fig. 2k ). These results suggest that tau acetylation inhibits tau-mediated stabilization of MTs. Tau acetylation on K280 detects tau pathology in Tg mouse models Genetic studies have shown that deletion of K280 (ΔK280) is associated with FTDP-17 familial tauopathy [11] . Although the disease mechanism associated with ΔK280 is not fully understood, in vitro analysis of ΔK280 demonstrated impaired MT assembly [22] and enhanced PHF aggregation [19] , [23] . Thus, K280 acetylation functionally mimics ΔK280, potentially by inhibition of electrostatic tau–MT interactions. To monitor K280 acetylation in brain tissue, a polyclonal antibody was generated against an acetylated K280 tau peptide. Double affinity purification yielded a site-specific acetylated K280 antibody (hereafter referred to as anti-ac-K280) that detected acetylated WT tau, but not a ΔK280 mutant tau demonstrated by in vitro and cell-based acetylation assays ( Supplementary Fig. S3 ). Ac-K280 positive cells were detected in the presence of active CBP, but not a catalytically inactive CBP mutant (CBP-LD). Moreover, expression of an HDAC6 small interfering RNA led to increased levels of ac-K280, further confirming the specificity of the anti-ac-K280 antibody and providing additional evidence that HDAC6 is a tau deacetylase ( Supplementary Fig. S3 ). Using anti-ac-K280, we probed tau acetylation in mouse brain by immunohistochemistry (IHC) using two tau Tg mouse models that recapitulate tau pathology and NFT formation: PS19 monogenic mice expressing P301S mutant tau [24] and PS19;PDAPP bigenic mice, which additionally express the APP V717F mutant transgene that accelerates NFT formation and enhances tau amyloidogenesis [25] . Monogenic PS19 tau Tg mice revealed moderate neuronal ac-K280 immunoreactivity in both cortex and hippocampus when compared with non-Tg mice, although abundant hyperphosphorylated tau was detected by AT8, a phospho-tau specific antibody ( Fig. 3a–d ). However, bigenic PS19;PDAPP mice showed profound age-dependent increase in ac-K280 tau pathology (see Supplementary Fig. S4 ), particularly in the hippocampus, in which the intensity of ac-K280 staining was increased relative to monogenic PS19 mice ( Fig. 3e,f ). Moreover, significant co-localization of ac-K280 immunoreactivity was observed with AT8 in tau inclusions of PS19;PDAPP bigenic mice using double-labelling IF ( Fig. 3g–i ). Ac-K280-positive tau inclusions were also detected by Thioflavin-S (ThS), which demonstrates that tau amyloid lesions are prominently acetylated in these mice ( Fig. 3j–l ). 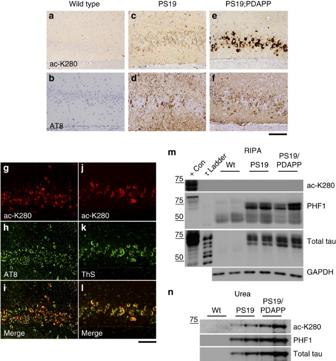Figure 3: Tau acetylation in Tg mouse models with tau pathology. (a–f) Immunohistochemistry (IHC) was used to analyse cortical sections from the following lines of mice: wild-type (WT) mice using anti-ac-K280 (a) or AT8 (b) antibodies, PS19 monogenic mice using anti-ac-K280 (c) or AT8 antibodies (d) and PS19;PDAPP bigenic mice using anti-ac-K280 (e) and AT8 antibodies (f). (g–i) Double-labelling immunofluorescence microscopy using anti-ac-K280 (g, red) and AT8 (h, green) antibodies on hippocampal sections from PS19;PDAPP mice showed extensive co-localization of acetylated and hyperphosphorylated tau inclusions (merged image,i). (j–l)Double labelling using anti-ac-K280 (j, red) and ThS (k, green), an amyloid-binding dye, also demonstrated co-localization of acetylated tau with Thioflavin-S-positive NFTs (merged image,l). Scale bars, 100 μm. (m,n) Sequential biochemical fractionation was performed on WT, PS19 and PS19/PDAPP mouse cortices using RIPA buffer followed by urea extraction. Soluble (m) and insoluble (n) extracted tau proteins were analysed by western blotting using anti-ac-K280, PHF-1 and total tau (T14/T46) antibodies. Figure 3: Tau acetylation in Tg mouse models with tau pathology. ( a–f ) Immunohistochemistry (IHC) was used to analyse cortical sections from the following lines of mice: wild-type (WT) mice using anti-ac-K280 ( a ) or AT8 ( b ) antibodies, PS19 monogenic mice using anti-ac-K280 ( c ) or AT8 antibodies ( d ) and PS19;PDAPP bigenic mice using anti-ac-K280 ( e ) and AT8 antibodies ( f ). ( g–i ) Double-labelling immunofluorescence microscopy using anti-ac-K280 ( g , red) and AT8 ( h , green) antibodies on hippocampal sections from PS19;PDAPP mice showed extensive co-localization of acetylated and hyperphosphorylated tau inclusions (merged image, i ). ( j–l) Double labelling using anti-ac-K280 ( j , red) and ThS ( k , green), an amyloid-binding dye, also demonstrated co-localization of acetylated tau with Thioflavin-S-positive NFTs (merged image, l ). Scale bars, 100 μm. ( m , n ) Sequential biochemical fractionation was performed on WT, PS19 and PS19/PDAPP mouse cortices using RIPA buffer followed by urea extraction. Soluble ( m ) and insoluble ( n ) extracted tau proteins were analysed by western blotting using anti-ac-K280, PHF-1 and total tau (T14/T46) antibodies. Full size image To determine the biochemical properties of acetylated tau, sequential extraction of normal and pathological tau from WT, PS19 and PS19/PDAPP mouse cortices was conducted using buffers of increasing strength. RIPA and urea solubilized brain extracts from mouse cortices were analysed by western blotting using anti-ac-K280, PHF-1 and total tau (T14/T46) antibodies. RIPA extracted cortical lysates contained the majority of the soluble tau pool, indicated by total tau levels ( Fig. 3m ). In contrast, anti-ac-K280 reactivity was undetectable in RIPA-solubilized extracts, but instead accumulated in the insoluble urea fraction ( Fig. 3n ). Consistent with the IHC analysis, immunoblotting also revealed increased ac-K280 levels in PS19; PDAPP bigenic compared with PS19 monogenic mice. Thus, tau acetylation is associated with biochemically insoluble, ThS-positive tau aggregates in tau Tg mouse models. Tau acetylation on K280 is found in a wide range of human tauopathies To investigate tau K280 acetylation in human neurodegenerative tauopathies, IHC was conducted on AD, corticobasal degeneration (CBD) and Pick's disease (PiD) cases (see Table 2 for human cases used in this study). These tauopathies share abundant filamentous tau pathology in affected brain regions, but differ in their patterns of insoluble tau isoforms with equal ratios of 3R/4R tau in AD, predominantly 4R-tau in CBD, and predominantly 3R-tau in PiD. Cortical brain sections of tauopathies were analysed using anti-ac-K280, which recognizes only 4R-tau isoforms as 3R-tau lacks K280 because of exon 10 alternative mRNA splicing. Remarkably, anti-ac-K280-positive NFTs and neuropil threads were prominently observed in AD cortex and resemble pathology detected by PHF-1 ( Fig. 4a–b ). CBD has extensive grey and white matter tau pathology of neuronal and glial tau inclusions, and anti-ac-K280 immunostained these tau pathologies similar to PHF-1 ( Fig. 4c–d ). Importantly, analysis of PiD inclusions containing primarily 3R-tau isoforms revealed no detectable anti-ac-K280 immunoreactivity ( Fig. 4e–f ), further validating anti-ac-K280 specificity. To determine whether acetylated tau is present within tau tangles, double IF microscopy revealed substantial co-localization of anti-ac-K280 and PHF-1 in all 4R-tau-specific tauopathies, including AD and CBD ( Fig. 4g–i and j–l , respectively). Moreover, ThS-positive NFTs present in AD brains also co-localized with anti-ac-K280 immunoreactive tau inclusions ( Fig. 4m–o ). To determine the scope of acetylated tau lesions in human disease, we extended these observations to a wide spectrum of tauopathies with 4R-tau pathology (see case demographics in Table 2 ). Indeed, anti-ac-K280-positive tau aggregates were observed in all other tauopathies examined including progressive supranuclear palsy, argyrophilic grain disease, tangle predominant senile dementia and Guam parkinsonism–dementia complex ( Supplementary Fig. S5 ). Thus, K280 acetylation is a feature found in a variety of human 4R or 3R/4R tauopathies including AD, but not 3R-tauopathies such as PiD. Table 2 Demographics of human tauopathy subjects used in this study. 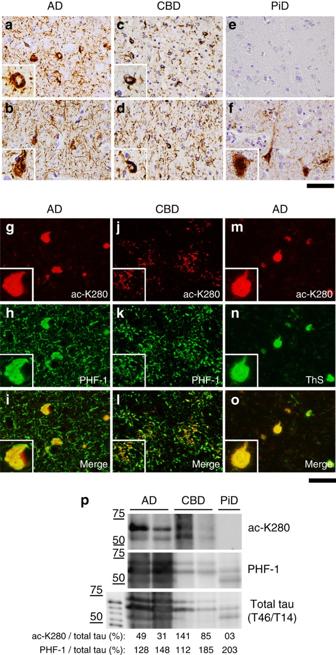Figure 4: Tau acetylation is associated with tau aggregation in human tauopathies. (a–f) Immunohistochemistry (IHC) was used to analyse cortical sections from the following tauopathies: Alzheimer's disease (AD) using anti-ac-K280 (a) or PHF-1 (b) antibodies, corticobasal degeneration (CBD) using anti-ac-K280 (c) or PHF-1 (d) antibodies and Pick's disease (PiD) using anti-ac-K280 (e) or PHF-1 (f) antibodies. Shown are representative images of tau inclusions with anti-ac-K280 and PHF-1 immunoreactivity. AD and 4R-tau predominant tauopathies (for example, corticobasal degeneration) were ac-K280 immuno-positive (a,c), whereas 3R-tau predominant Pick's disease was negative (e). (g–l) Double-labelling immunfluorescence was performed on cortical sections from AD using anti-ac-K280 (g, red) and PHF-1 (h, green) antibodies (merged image,i). Similar analysis was performed using sections from CBD using anti-ac-K280 (j, red) and PHF-1 (k, green) antibodies (merged image,l). (m–o)Double labelling of neurofibrillary tangles (NFTs) in AD cortex was detected using anti-ac-K280 (m, red) and Thioflavin S (n, green) and the corresponding merged image is shown ino. Insets represent ×60 magnification. Scale bar, 50 μm. (p) Biochemical isolation of enriched PHFs was performed on frontal cortex from indicated tauopathies and solubilized PHF-tau was analysed by immunoblotting using anti-ac-K280, PHF-1 and total tau (T14/T46) antibodies. Ac-K280 and PHF-1 immunoreactivity was quantified using Multi Guage v2.3 and raw intensities are represented below as percent modified tau species/total tau intensities to compare acetylated versus phosphorylated tau ratios. Full size table Figure 4: Tau acetylation is associated with tau aggregation in human tauopathies. (a–f ) Immunohistochemistry (IHC) was used to analyse cortical sections from the following tauopathies: Alzheimer's disease (AD) using anti-ac-K280 ( a ) or PHF-1 ( b ) antibodies, corticobasal degeneration (CBD) using anti-ac-K280 ( c ) or PHF-1 ( d ) antibodies and Pick's disease (PiD) using anti-ac-K280 ( e ) or PHF-1 ( f ) antibodies. Shown are representative images of tau inclusions with anti-ac-K280 and PHF-1 immunoreactivity. AD and 4R-tau predominant tauopathies (for example, corticobasal degeneration) were ac-K280 immuno-positive ( a , c ), whereas 3R-tau predominant Pick's disease was negative ( e ). ( g–l ) Double-labelling immunfluorescence was performed on cortical sections from AD using anti-ac-K280 ( g , red) and PHF-1 ( h , green) antibodies (merged image, i ). Similar analysis was performed using sections from CBD using anti-ac-K280 ( j , red) and PHF-1 ( k , green) antibodies (merged image, l ). ( m–o) Double labelling of neurofibrillary tangles (NFTs) in AD cortex was detected using anti-ac-K280 ( m , red) and Thioflavin S ( n , green) and the corresponding merged image is shown in o . Insets represent ×60 magnification. Scale bar, 50 μm. ( p ) Biochemical isolation of enriched PHFs was performed on frontal cortex from indicated tauopathies and solubilized PHF-tau was analysed by immunoblotting using anti-ac-K280, PHF-1 and total tau (T14/T46) antibodies. Ac-K280 and PHF-1 immunoreactivity was quantified using Multi Guage v2.3 and raw intensities are represented below as percent modified tau species/total tau intensities to compare acetylated versus phosphorylated tau ratios. Full size image To demonstrate acetylated tau is present in PHFs of human tauopathies, we extracted PHFs from cortical regions of AD, CBD and PiD brains [5] , [8] and immunoblotted using anti-ac-K280, PHF-1 and T14/T46 (total tau) antibodies ( Fig. 4p ). Prominent PHF-tau isoforms were detected with PHF-1 and T14/T46 antibodies, confirming isolation of insoluble and hyperphosphorylated 4R/3R-tau (AD), 4R-tau (CBD) or 3R-tau (PiD) species. Consistent with the above IHC results, anti-ac-K280 detected 4R tau isoforms in AD and CBD cases, but not the 3R-tau isoforms in PiD. Furthermore, acetylation of normal soluble tau was never observed. These results are consistent with more prominent acetylation occurring specifically on pathologically insoluble, aggregated PHF-tau species. This study demonstrates tau acetylation as a post-translational modification that may regulate normal tau function and suggests a role in pathological tau aggregation in AD and related tauopathies. Increased tau acetylation on K280 could impair tau interactions with MTs and provide increased pools of cytosolic tau available for pathological PHF aggregation. Consistent with this, K280, located in the inter-repeat region, was identified previously as one of three lysine residues most critical in modulating tau–MT interactions [22] . Moreover, K280 acetylation was not observed in tau fibrils assembled from recombinant T40 because this residue is buried within the fibril core. Thus, our data support the notion that K280 acetylation occurs before tau fibrillization into PHFs and therefore is likely a pathological event. Indeed, K280 acetylation was detected in all 4R- and 3R/4R-tauopathies that we examined, but was absent in 3R predominant PiD brains or soluble tau fractions of normal control samples. Acetylation of tau aggregates was associated with hyperphosphorylated, ThS-positive tau inclusions in both Tg mouse models and human tauopathies. This implies that negative regulation of tau function could occur via phosphorylation and acetylation events alone or in combination. Tau is extensively phosphorylated on at least 25 distinct serines/threonines residues, most of which are outside the MT-binding repeat region. In contrast, tau acetylation in cells was specifically detected on four lysines, three of which are located within the MT-binding repeats. Thus, tau acetylation and phosphorylation may represent specific modifications required to dynamically regulate tau function. One possibility is that increased tau phosphorylation could facilitate tau acetylation within the MT repeat domain to further impair tau binding to MTs, suggesting complex regulation of tau–MT dynamics. A more comprehensive analysis of acetylated and phosphorylated sites in diseased brains could provide insight into the potential cooperative regulation of tau post-translational modifications during disease pathogenesis. K280 resides in the double lysine motif, 275 VQIINKK 281 , which is critical for MT binding. Indeed, this motif is conserved in other tau family members including MAP2 and MAP4, indicating reversible acetylation could represent a conserved mechanism to regulate the MT-binding activity of other MAPs in addition to tau. Although protein acetylation has been extensively studied in the context of histones and gene transcription, proteomics approaches have identified acetylated proteins in the cytoplasm and other organelles [26] . Several acetyl-transferases and deacetylases (HDACs) are localized to the cytoplasm and MTs [27] , [28] , suggesting acetylation may represent a general mechanism to regulate cytoskeletal dynamics and coordinate cytoplasmic signalling events. Finally, our IHC and biochemical studies suggest that K280 acetylation may be more disease specific than phosphorylated tau in tauopathies. Thus, monitoring acetylated tau levels may represent a potential biomarker for the diagnosis of AD and related neurodegenerative tauopathies. Moreover, the identification of tau acetylation in tauopathies provides a framework for both biomarker development and for therapeutic targeting of tauopathies via the acetylation/deacetylation machinery. Plasmids and cell culture WT-CBP and CBP-LD inactive mutants as well as WT-HDAC6 and HDAC6-H803A enzyme-inactive mutant expression plasmids were kindly provided by Dr Tso-Pang Yao (Duke University). The longest human tau isoform (designated Tau-T40) was cloned into pCDNA5/TO vector (Invitrogen) and site-directed mutagenesis (Quikchange kit; Stratagene) was used to create K→Q or K→R mutations at residues K163, K280, K281, K369 as indicated. Indicated plasmids were transfected into either QBI-293 cells or stably expressing HEK-T40 cells using Fugene (Roche). HEK-T40 cells were generated using 293 T-Rex cells (Invitrogen) transfected with pcDNA5/TO WT-T40 and selected with 200 μg ml −1 of hygromycin and 5 μg ml −1 blasticidin. Resistant clones were isolated from single cells and screened for tau expression by IF and immunoblotting. IF and MT bundling analysis of transiently transfected QBI-293 cells were performed as previously described [21] . HDAC6 siRNA (Invitrogen) sequence was as follows: 5′-AAAGUUGGAACUCUCACGGUGCAGC-3′ and was transfected using RNAi Max reagent (Invitrogen) following manufacturer protocols. Monoclonal antibodies used for western analysis were as follows: T46 (1:1000), T14 (1:1000), PHF-1 (1:1000) and AT-8 (1:500). Polyclonal antibodies used were as follows: ac-K280 (1:1000), anti-acetyl-lysine (1:1000, Cell Signaling), E10 (1:500), HDAC6 (1:1000, Santa Cruz). Recombinant tau in vitro methods Tau K18 protein was either mock acetylated or acetylated in vitro using acetyl-CoA substrate as indicated in legend to Figure 1 . Acetylation reaction samples were pooled together, concentrated to 1 ml using Amicon Ultra centrifugal filter units (Millipore Corporation) and ten-fold diluted with 100 mM sodium acetate buffer (pH 7.0) three times followed by concentration to 100 μl of concentrated tau protein. Protein concentrations were determined using the bicinchoninic acid protein assay (Pierce) with bovine serum albumin as the standard. Acetylated K18 and mock-treated K18 were assessed by a light-scattering assay as described in legend to Figure 1c . For fibrillization reactions, 10–20 μM K18 proteins were incubated at 37 °C with equal molar ratio of heparin in 100 mM sodium acetate buffer (pH 7.0) containing 2 mM dithiothreitol (DTT). The extent of fibrillization was assessed at different time points by ThT fluorescence assay, sedimentation analysis and negative staining EM as described in the legend to Figure 1 . For ThT fluorescence assay, ThT diluted in 100 mM glycine buffer (pH 8.5) was added and fluorometric readings were taken at 450 nm (excitation) and 510 nm (emission). The assay was performed in triplicate. For sedimentation test, 40 μl fibrillization mixtures were centrifuged at 100,000 g for 30 min at 4 °C to separate fibrils soluble supernatant fractions. Pellets were washed once with 100 mM sodium acetate buffer (pH 7.0) and resuspended in 40 μl of the same buffer. Equal volume of fractions were analysed by 15% SDS–PAGE gels followed by Coomassie staining. For negative staining EM, 6 μl of fibrillization mixture from each time point were placed on 300 meshed Formvar/ carbon film-coated copper grids (Electron Microscopy Sciences) for 3 min, washed twice with 50 mM Tris buffer (pH 7.6) for 5 min each, stained with 10–15 drops of 2% uranyl acetate and visualized with Jeol 1010 transmission electron microscope (Jeol). Peptide and antibody generation Polyclonal anti-acetyl tau K280 antibodies were generated using the acetylated tau peptide C-QIINKKLDLSN containing K280 acetylation to immunize rabbits (Pocono Rabbit Farm and Laboratory). Double affinity purification was performed using native and acetylated peptides sequentially using Sulfolink columns (Pierce Biotechnology). Site specificity of ac-K280 was confirmed in vitro and in cells using tau proteins lacking residue K280 ( Supplementary Fig. S3 ). Histology and IHC Tissue preparation and IHC were performed on monogenic PS19 and bigenic PS19;PDAPP transgenic mice at 4, 8 and 11 months of age as described. Mice were anaesthetized and transcardially perfused with phosphate buffer saline, pH 7.0 in accordance with protocols approved by the Institutional Animal Care and Use Committee of the University of Pennsylvania. Brains were surgically removed and fixed in 4% neutral-buffered formalin. Coronal slabs were fixed in neutral-buffered formalin and paraffin embedded. Paraffin blocks were sectioned at 6 μm through the entire block. Tissues sections were stained using a Polymer horseradish peroxidase detection system (Biogenex) and automatically stained using the i6000 Automated Staining System (Biogenex). For human studies, fixed, paraffin-embedded tissue blocks were obtained from the Center for Neurodegenerative Disease Research Brain Bank at the University of Pennsylvania. Consent for autopsy was obtained from legal representatives for all subjects in accordance with local institutional review board requirements. Briefly, fresh tissues from each brain were fixed with 70% ethanol in 150 mmol l −1 NaCl, infiltrated with paraffin and cut into 6-μm serial sections. IHC was performed using the avidin–biotin complex detection system (Vector Laboratories) and 3,3′-diaminobenzidine. Briefly, sections were deparaffinized and rehydrated, antigen retrieval was done by incubating section in 88% formic acid, endogenous peroxidases were quenched with 5% H 2 O 2 in methanol for 30 min and sections were blocked in 0.1 mol l −1 Tris with 2% fetal bovine serum for 5 min. Primary antibodies were incubated for either 1 or 2 h at room temperature or overnight at 4 °C. The following primary antibodies were used for IHC analysis: affinity purified rabbit anti-acetyl-tau (ac-K280; 1:250-1:2000), mouse anti-phospho-tau Ser202/Thr205 (AT8; 1:15,000), mouse anti-phospho-tau Ser396/Ser404 (PHF-1; 1:1000). After washing, sections were sequentially incubated with biotinylated secondary antibodies for 1 h and avidin–biotin complex for 1 h. Bound antibody complexes were visualized by incubating sections in a solution containing 100 mM TrisHCl, pH 7.6, 0.1% Triton X-100, 1.4 mM diaminobenzidine, 10 mM imidazole and 8.8 mM H 2 O 2 . Sections were then lightly counterstained with hematoxylin, dehydrated and coverslipped. Double-labelling IF Double-labelling IF analyses were performed using Alexa Fluor 488- and 594-conjugated secondary antibodies (Molecular Probes), treated for autofluorescence with Sudan Black solution and coverslipped with Vectashield mounting medium (Vector Laboratories). Double-labelling ThS and IF was performed through sequential methods initially staining sections with ThS followed by IF. Briefly, sections were deparaffinized and hydrated to dH 2 O, immersed in PBS pH7.3 for 5 min followed by immersion in 0.05% KMnO 4 /PBS for 20 min. Sections were rinsed in PBS and destained in 0.2% K 2 S 2 O 5 /O.2% oxalic acid/PBS and immersed in 0.0125% ThS/40% EtOH/60% PBS and differentiated in 50% EtOH/50%PBS for 10–15 min. After differentiation, sections were incubated with rabbit anti-ac-K280 overnight at 4 °C using standard IF techniques. Digital images were obtained using an Olympus BX 51 microscope (Olympus) equipped with bright-field and fluorescence light sources using a ProgRes C14 digital camera (Jenoptik AG) and Adobe Photoshop, version 9.0 (Adobe Systems) or digital camera DP71 (Olympus) and DP manager (Olympus). Biochemical extraction PHFs were isolated from normal and tauopathy brains as previously described [29] . Briefly, grey matter was homogenized in 3 vol per g of cold High Salt RAB buffer (0.75 M NaCl, 100 mM Tris, 1 mM EGTA, 0.5 mM MgSO 4 , 0.02 M NaF, 2 mM DTT, pH 7.4). All buffers were supplemented with protease inhibitor cocktail, phosphatase inhibitor and HDAC inhibitors (2 μM TSA and 10 mM nicotinamide). Homogenates were incubated at 4 °C for 20 min to depolymerize MTs, then, centrifuged at 100,000 g for 30 min at 4 °C. Pellets were re-homogenized and centrifuged in 3 vol per g of cold High Salt RAB buffer. Resultant pellets were homogenized in 5 vol per g of cold PHF extraction buffer (10 mM Tris pH 7.4, 10% sucrose, 0.85 M NaCl, 1 mM EGTA, pH 7.4) and centrifuged at 15,000 g for 20 min at 4 °C. Sarkosyl was added to the supernatant (1% final concentration) and incubated at 4 °C overnight followed by centrifugation for 30 min at 100,000 g to generate crude PHF-tau fractions, which were solubilized by formic acid extraction. Fractionation of mouse cortices was performed by sequential extraction using buffers of increasing strength. Brain tissue was homogenized in 5 vol per g of low-salt buffer (10 mM Tris pH 8.0, 2 mM EDTA, 1 mM DTT) and centrifuged at 100,000 g for 30 min to generate low-salt fractions. Myelin floatation was performed on pellets re-extracted in low-salt buffer supplemented with 20% sucrose. Resulting pellets were re-extracted in 5 vol per g of RIPA buffer (50 mM Tris pH 8.0, 150 mM NaCl, 1%NP-40, 5 mM EDTA, 0.5% sodium deoxycholate, 0.1%SDS). Finally, resultant insoluble pellets were extracted in 1 vol per g of tissue in urea buffer (7 M urea, 2 M Thiourea, 4% CHAPS, 30 mM Tris, pH 8.5). Soluble and insoluble fractions were analysed by SDS–PAGE electrophoresis and western blotting using the indicated antibodies to detect total, acetylated or phosphorylated tau proteins. How to cite this article: Cohen, T. J. et al . The acetylation of tau inhibits its function and promotes pathological tau aggregation. Nat. Commun. 2:252 doi: 10.1038/ncomms1255 (2011).